Sources of heterogeneous variability and trends in Antarctic sea-ice While the Northern Hemisphere sea-ice has uniformly declined over the past several decades, the observed sea-ice in the Southern Hemisphere has exhibited regions of increase and decrease. Here we use a comprehensive set of ocean–sea-ice simulations (1990–2007) to elucidate the drivers of the observed heterogeneous sea-ice trends. We show wind variability is an important determinant of the heterogeneous pattern of the variability and trends in Southern Hemisphere sea-ice. Only in the West Pacific region does Southern Annular Mode wind forcing contribute significantly to the trend in sea-ice duration. El Niño Southern Oscillation wind forcing contribution to the sea-ice duration trend is confined to the Atlantic and Pacific. In the Indian Ocean, weather is a significant driver of the sea-ice duration trend. Only in the East Pacific region is wind forcing alone insufficient to give rise to the observed sea-ice decline and must be augmented by warming to reproduce the observations. The Southern Ocean plays an important role in climate [1] and carbon cycling [2] . The Southern Hemisphere sea-ice modulates the air–sea exchange of heat, freshwater and carbon, as well as the surface albedo [3] . Since sea-ice can influence climate, understanding the drivers of heterogeneity in the variability and trends in Antarctic sea-ice is necessary to projecting future climate change. The temporal variation in sea-ice extent both over the seasonal and multi-year timescales is associated with climate variability and long-term climate change. An interesting aspect of Southern Hemisphere sea-ice is its contrasting behaviour in recent decades to Northern Hemisphere sea-ice [4] . In the Northern Hemisphere, observations reveal that the sea-ice area, extent and volume have declined rapidly during recent decades [5] , [6] , with the change in extent being −5% per decade since 1985 (ref. 5 ). This large reduction in sea-ice extent is thought to be associated with global warming, such that decreases in sea-ice amplify Arctic warming through surface albedo feedback [7] . While the Northern Hemisphere has experienced a substantial decline in sea-ice, total Southern Hemisphere sea-ice has exhibited a modest increase over the satellite observation period (by 2% per decade since 1985) [8] . The satellite observations of Southern Hemisphere sea-ice also reveal distinct regional behaviour, with decreases in concentration and duration in the western Antarctic Peninsula and southern Bellingshausen Sea but increases in the Ross and Amundsen Seas [9] , [10] , [11] . The spatial structure to sea-ice trends [12] , [13] is similar to the Antarctic Dipole pattern [14] . The Antarctic Dipole pattern also characterizes the leading mode of interannual variability in Southern Hemisphere winter sea-ice cover [14] , reflecting the out-of-phase relationship between the Atlantic and Central Pacific sectors of the Southern Hemisphere. Against the background of global warming, the expansion of Antarctic sea-ice is a curious phenomenon requiring explanation. Recently, observations and modelling have highlighted the importance of wind variability in accounting for the behaviour of Southern Hemisphere sea-ice [10] , [15] , [16] , [17] , [18] , [19] . Originally, it was argued that trends in dynamics and thermodynamics linked to local winds were responsible for producing the regional sea-ice trends in most sectors of the Southern Ocean [16] . More recently, it has been suggested [20] that the largest autumn concentration trends were caused by trends in the temporal derivative of sea-ice concentrations during spring, complicating the direct link between wind anomalies and autumn sea-ice trends. Such results are consistent with observations that anomalies in autumn ice advance are better correlated with patterns in the preceding spring than with those in the subsequent spring [13] . This correlation amplifies the trend in sea-ice duration and suggests ice albedo and ocean heat uptake feedbacks [13] . The role of the winds, coupled with the lag response in Southern Hemisphere sea-ice, indicates the complexity of the atmosphere–ocean–sea-ice system. Model simulations provide a way to help elucidate the link between climate variability and sea-ice variability and trends. As previous studies have suggested that the Southern Annular Mode (SAM) [21] , [22] , the El Niño Southern Oscillation (ENSO) [23] , [23] and the weather [24] , [25] may all be important factors in sea-ice variability and trends, a study to assess the dominant drivers is needed. 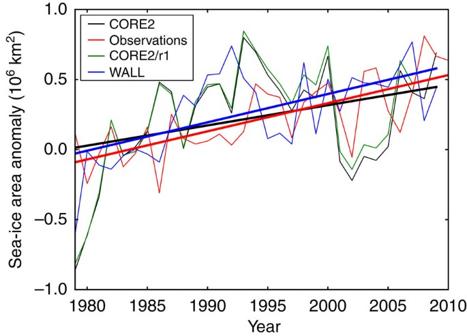Figure 1: Annual sea-ice area anomaly. The CORE2 simulation is shown by the thin green and black lines, the observations26by the thin red line and WALL simulation by the thin blue line. The thick straight lines represent the linear trends over the period. The two CORE2 lines (green and black) show the differences in two repeated rounds of the CORE2 forcing, used to illustrate how the initial ocean state influences the sea-ice trend. In this work, we present simulations to assess the regional response of sea-ice to SAM, ENSO and atmospheric weather forcings; the experiments are summarized in Table 1 , with details given in the Methods section. We consider wind variability due to ENSO, SAM and atmospheric weather separately, as well as the response to total wind variability in the absence of interannual surface temperature forcing (WALL). Total wind variability is not equal to the sum of ENSO, SAM and weather winds because a substantial amount of the wind variability is not associated with these three components. We use an additional simulation (Coordinated Ocean ice Reference Experiment version 2 (CORE2)) to elucidate the potential for interactions of the wind fields with atmospheric surface air temperature changes. Our simulations show wind variability is an important determinant of the heterogeneous pattern of the variability and trends in Southern Hemisphere sea-ice. With SAM wind forcing making a significant contribution to sea-ice duration trends in the East Pacific and ENSO wind forcing making a significant contribution to sea-ice duration trends in the Atlantic and Pacific. Weather is a significant contributor to sea-ice duration trend around the hemisphere. Only in the East Pacific region is wind forcing alone insufficient to give rise to the observed sea-ice decline and must be augmented by warming to reproduce the observed trend. Table 1 Brief description of the model simulations. Full size table Sea-ice interannual variability To assess the simulated Southern Hemisphere sea-ice behaviour, we compare the annual sea-ice area anomaly obtained from the CORE2 simulation (which applies interannually varying atmospheric forcing comprising winds, atmospheric temperatures and precipitation) with satellite observations [26] ( Fig. 1 ). At the hemispheric scale, the simulation reproduces the increasing trend in annual sea-ice area over the 1979–2008 period; the simulated trend is 1.5 × 10 11 m 2 per decade increase, and the observed trend is 2.0 × 10 11 m 2 per decade increase. Two repeated rounds of CORE2 forcing were applied to ascertain whether the trend is sensitive to the initial ocean state, and it appeared not to be (compare the green and black lines in Fig. 1 ). We also compute the hemispheric trends from the component simulations, which show weather simulation—high frequency (WHF), ENSO, SAM and ENSO+SAM trends are weak: 2.2 × 10 10 , 1.8 × 10 10 , 1.65 × 10 10 m 2 per decade and 3.6 × 10 10 m 2 per decade, respectively. However, the simulation with just wind variability (WALL) does produce a larger trend, 2.02 × 10 11 m 2 per decade, than the CORE2 simulation and is more consistent with the observations. Including the variability in the CORE2 air temperature significantly reduces the hemispheric increase in sea-ice area. Figure 1: Annual sea-ice area anomaly. The CORE2 simulation is shown by the thin green and black lines, the observations [26] by the thin red line and WALL simulation by the thin blue line. The thick straight lines represent the linear trends over the period. The two CORE2 lines (green and black) show the differences in two repeated rounds of the CORE2 forcing, used to illustrate how the initial ocean state influences the sea-ice trend. Full size image Southern Hemisphere sea-ice drift is linked to local winds and has made an important contribution to sea-ice concentration trends around much of West Antarctica over the 1992–2010 period [16] . We use vector correlation over the approximate period of satellite-tracked sea-ice motion observations (1990–2008) to quantify the effect winds have on ice motion, both through direct wind stress and through the forcing from ocean stress and sea-surface tilt that is correlated with local winds. 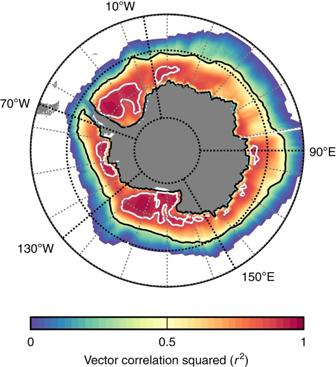Figure 2: Vector correlation between the April–October time series of the winds and the sea-ice drift for the 1990–2007 period. In the figure a significant correlation occurs for values >0.4, denoted by the black contour line. The white contour line shows the 0.9 isopleth. Figure 2 shows the vector correlation between the interannual time series of April–October mean ice motion and CORE2 winds (see the Methods section). Areas of low correlation are regions where ice motion is not attributed to the winds because of modifications by internal stresses. The simulated hemispheric average correlation is r 2 =0.65, slightly greater than the observed value ( r 2 =0.52) [16] . Consistent with the observations, the simulation shows large areas in the Atlantic and Pacific away from the continent that have high correlation values, whereas in the Indian Ocean the correlation is generally less but with several isolated areas with high values ( Fig. 2 ). Generally, the simulation has greater correlation than is estimated from the observation [16] , particularly in the Indian Ocean. The greater correlation of the simulation than is observed may reflect the simulation lacking errors in ice tracking and having ice dynamics consistent with atmospheric forcing [16] . The greater correlation may also reflect unrealistic behaviour in the simulated sea-ice. The simulation shows a clear link between winds and sea-ice behaviour, again consistent with the observations, but perhaps with a tendency to underestimate the modification of ice motion by internal stresses. Figure 2: Vector correlation between the April–October time series of the winds and the sea-ice drift for the 1990–2007 period. In the figure a significant correlation occurs for values >0.4, denoted by the black contour line. The white contour line shows the 0.9 isopleth. Full size image To assess the simulated variability in winter sea-ice concentration (defined as the average ice concentration during the months of March–October), we compare the s.d. in winter sea-ice concentration obtained from the CORE2 simulation ( Fig. 3a ) with that of the satellite observations [26] ( Fig. 3b ). The simulated variability is similar in magnitude and pattern to the observations; both show greatest variability in the Pacific sector around 120°W and near the Antarctic Peninsula. This is the region where mean sea level pressure shows the greatest variability [27] . Further, as seen in Fig. 4 , the simulated variability in winter sea-ice extent (defined as the latitude going south from the equator where the winter sea-ice concentration becomes >15%) is similar to that shown by satellite observations. Over the observational period, the simulated winter sea-ice extent was found to be significantly correlated with the observations ( r =0.45, P -value<0.0001). For the correlation calculation, the observations in Fig. 4b were regrid in space and time onto the model grid and then correlated with the simulated values ( Fig. 4a ). 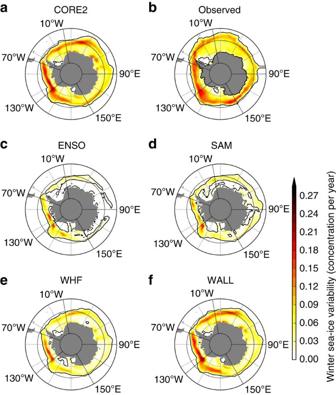Figure 3: Standard deviation in winter sea-ice concentrations. For (a) CORE2 simulation, (b) satellite observations26, (c) ENSO component simulation, (d) SAM component simulation, (e) high-frequency weather forcing (WHF) simulation and (f) all wind forcing (WALL) simulation. Figure 3: Standard deviation in winter sea-ice concentrations. For ( a ) CORE2 simulation, ( b ) satellite observations [26] , ( c ) ENSO component simulation, ( d ) SAM component simulation, ( e ) high-frequency weather forcing (WHF) simulation and ( f ) all wind forcing (WALL) simulation. 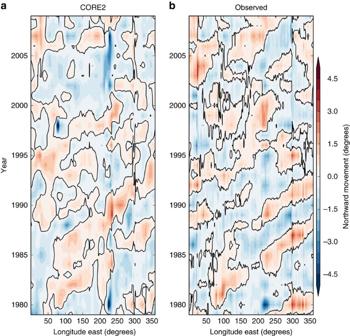Figure 4: Hovmoller plot around Antarctica showing north–south departures in winter sea-ice extent from the 1979 to 2007 averaged position. The north–south departures, in degrees latitude, are shown for (a) the CORE2 simulation and (b) the satellite observations26. Full size image Figure 4: Hovmoller plot around Antarctica showing north–south departures in winter sea-ice extent from the 1979 to 2007 averaged position. The north–south departures, in degrees latitude, are shown for ( a ) the CORE2 simulation and ( b ) the satellite observations [26] . Full size image The observed winter sea-ice extent can vary by ±5° latitude, and there is the appearance of a wave-like propagation from the Pacific to the Atlantic sector in the 1980s and early 1990s [28] ( Fig. 4b ), with a propagation speed of ∼ 40° longitude per year. Figure 4a shows that the CORE2-simulated winter sea-ice extent variability has a similar magnitude to the observations, and also exhibits a wave-like propagation through the 1980s and early 1990s. After 1995, the wave-like structure is largely absent from the simulation, consistent with the observations [29] . The significant correlation between and similar magnitude of the CORE2-simulated and observed winter sea-ice extent gives us some confidence that the simulation is capturing key features (including regional variations) of Southern Hemisphere sea-ice variability that arise in response to atmospheric forcing. To help discern the factors that drive winter sea-ice variability, we separate the atmospheric wind forcing into components due to low-frequency SAM and ENSO variability and a component due to high-frequency weather forcing (WHF, see the Methods section and Table 1 for details). For SAM and ENSO, we investigate their impact on winter sea-ice variability both separately and together (ENSO+SAM). In the SAM and ENSO simulations, significant winter sea-ice variability is confined to the Pacific sector, with weak variability in the Atlantic and Indian Ocean sectors ( Fig. 3c,d ). In contrast, the WHF simulation produces more variability, and significant variability is evident in all three sectors of the Southern Ocean ( Fig. 3e ). In the WHF simulation, the greatest variability occurs in the Pacific sector, at the same location as in the CORE2 simulation and the observations. The WHF simulation also shows substantial winter sea-ice variability in the Atlantic sector. Overall, the pattern of variability in the WHF simulation is highly correlated with that in the CORE2 simulation ( r =0.5, P -value<0.001), and its magnitude of variability is ∼ 75% of the magnitude in the CORE2 simulation. By including all the wind variability (WALL), both the magnitude and pattern of variability ( Fig. 3f ) look similar to the observations. Atmospheric weather plays an important role in multi-year winter sea-ice variability. The importance of atmospheric weather is consistent with atmospheric cyclone analysis in the Southern Hemisphere, which indicates that areas of stronger polar cyclones are also areas of maximum sea-ice displacement [25] . While the winter sea-ice response can occur through the local impact of weather on ice growth and transport [25] , this is not the only mechanism. Using nominal year forcing (Coordinated Ocean ice Reference Experiment version 1 (CORE1)), we have previously identified an intrinsic decadal mode of variability in the Southern Ocean, which links thermocline variability with sea-ice variability [30] , [31] . The intrinsic decadal Southern Ocean sea-ice variability, excited by stochastic wind variability, was substantially amplified (by coherence resonance effects) when the coherent variability of the observed synoptic-scale weather was used to force the ocean [31] . By exciting the intrinsic mode, the atmospheric weather generates additional variability in the winter sea-ice, which can then give rise to multi-year variability. Sea-ice duration trends For the period 1990–2007, the CORE2 simulation produced a trend in sea-ice duration (calculated as the number of days on which sea-ice concentration exceeded 10% cover) with prominent spatial heterogeneity ( Fig. 5a ). The time period for calculating the trend was chosen to match the duration and approximate period of satellite-tracked sea-ice motion observations (1992–2010). Over this period, observations show that ice-motion trends are dominated by winds, and that winds contribute significantly to ice-concentration trends through both dynamic and thermodynamic effects [16] . Consistent with the observations, the CORE2 simulation reveals spatial heterogeneity in the Antarctic sea-ice duration ( Fig. 5a,b ). Based on the heterogeneous nature of observed sea-ice duration trends, we divide the Southern Ocean into five distinct sectors ( Fig. 6 ). Within each of these sectors the observed duration trends are significant at the P <0.001 level. In the following, we describe the observed trend in each sector and use the component simulations to explore their contribution to the sector trends. While sea-ice trends reflect the combined response of all atmospheric forcings, the different components of the atmospheric forcing acting alone may not have an expression in all sectors. To help assess the importance of the different atmospheric forcings we correlated the observed trends at each grid point in a sector with the trends of the various simulations. 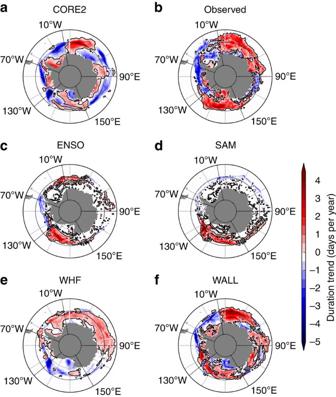Figure 5: Trends in sea-ice duration over the 1990–2007 period in days per year. For (a) CORE2 simulation, (b) satellite observations26, (c) ENSO component simulation, (d) SAM component simulation, (e) high-frequency weather forcing (WHF) simulation and (f) all wind forcing simulation (WALL). In (b) the green contour lines denote those trends with significance at theP<0.05 level. Figure 5: Trends in sea-ice duration over the 1990–2007 period in days per year. For ( a ) CORE2 simulation, ( b ) satellite observations [26] , ( c ) ENSO component simulation, ( d ) SAM component simulation, ( e ) high-frequency weather forcing (WHF) simulation and ( f ) all wind forcing simulation (WALL). In ( b ) the green contour lines denote those trends with significance at the P <0.05 level. 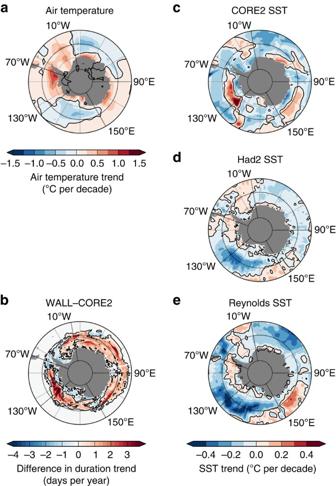Figure 6: For the 1990–2007 period, trends in annual mean air and sea-surface temperatures and in sea-ice duration. (a) The trend in annual mean air temperature (°C per decade) from the CORE2 forcing data; (b) the difference in sea-ice duration trends (days per year) between the WALL simulation and the CORE2 simulation. For comparison, the sea-surface temperature trend (°C per decade) from (c) the CORE2 simulation; (d) the observationally derived HadSST2 data set33; (e) the observationally derived Reynolds SST data set34. Full size image Figure 6: For the 1990–2007 period, trends in annual mean air and sea-surface temperatures and in sea-ice duration. ( a ) The trend in annual mean air temperature (°C per decade) from the CORE2 forcing data; ( b ) the difference in sea-ice duration trends (days per year) between the WALL simulation and the CORE2 simulation. For comparison, the sea-surface temperature trend (°C per decade) from ( c ) the CORE2 simulation; ( d ) the observationally derived HadSST2 data set [33] ; ( e ) the observationally derived Reynolds SST data set [34] . Full size image The West Atlantic sector (70°W to 10°W) shows a prominent declining trend in observed sea-ice duration ( Fig. 5b ). The CORE2 simulation ( Fig. 5a ) is in agreement with the observations, showing declining sea-ice duration in this sector, but the decline is much greater than is observed. Here, acting on its own: weather forcing increases sea-ice duration ( Fig. 5e ); ENSO forcing also produces a weak increasing trend ( Fig. 5c ); while SAM forcing generates no significant trend ( Fig. 5d ). None of the three components acting alone captures the observed trend. However, considering all the wind variability (WALL) in this sector yields a declining trend ( Fig. 5f ) that is most similar to the observations ( r =0.28, P <0.001). The East Atlantic–West Indian sector (between 10°W and 90°E) shows a generally increasing trend in observed sea-ice duration ( Fig. 5b ). The CORE2 simulation ( Fig. 5a ) produces a similar increasing trend in the western half of the sector (10°W to 40°E), but between 40°E and 90°E it shows a declining sea-ice duration that is not present in the observations. Compared with CORE2, the WALL simulation ( Fig. 5f ) yields better agreement with the observations ( r =0.34, P <0.001). From the component simulations, atmospheric weather produces an increasing sea-ice duration trend in the entire sector that is most similar to the observations ( r =0.25, P <0.001, Fig. 5e ). ENSO forcing produces an increasing trend but only west of 30°E ( Fig. 5c ), and SAM ( Fig. 5d ) produces no trend. In this sector as revealed by the WALL simulation, the wind variability that is not related to ENSO, SAM and WHF makes a substantial contribution to the sea-ice duration trend. The East Indian sector (between 90°E and 150°E) shows a weak declining trend in observed sea-ice duration ( Fig. 5b ). The CORE2-simulated trend ( Fig. 5a ) is more complex, with an increasing trend along the Antarctic Continent and a declining trend offshore that is similar to the observations. In this sector, the observed declining trend is weak, and the WHF simulation produces a similar declining sea-ice duration trend ( r =0.2, P <0.001; Fig. 5e ). In contrast, ENSO forcing alone produces no trend and SAM forcing alone produces a weak increasing trend ( Fig. 5c,d ). The West Pacific sector (150°E to 130°W) shows a prominent increasing trend in observed sea-ice duration ( Fig. 5b ). The CORE2 simulation ( Fig. 5a ) produces a much weaker increasing trend in sea-ice duration and lacks some of the increasing trends in the Ross Sea (180°E). In this sector, the WALL simulation better reproduces the observed trend than the CORE2 simulation. Both the ENSO and the SAM forcing acting on their own produce positive trends in this sector, making an important contribution to the observed trend. The increase in sea-ice duration is best represented by the combined SAM and ENSO forcings ( r =0.31, P <0.001; Fig. 5c,d ). In contrast, weather forcing produces negative trends ( Fig. 5e ) and explains the negative trend in the Ross Sea in the WALL and CORE2 simulations ( Fig. 5a,f ). The East Pacific sector (130°W to 70°W) shows a strong decreasing trend in observed sea-ice duration ( Fig. 5b ), with the trend being most significant along the Antarctic Peninsula and into the central Pacific [13] . Both the SAM and ENSO simulations ( Fig. 5c,d ) produce declines in sea-ice duration along the Antarctic Peninsula; however, the magnitudes are much less than observed. From the component forcings the strong decrease in sea-ice duration is best captured by ENSO forcing ( r =0.31, P <0.001; Fig. 5c ), but an additional mechanism is needed to produce the magnitude of the observed decline. These results agree with recent analysis [32] showing that ENSO and SAM explained less than one-third of the total trend in Southern Hemisphere sea-ice. To understand the response in this sector, we need to examine in more detail the distinctions between the CORE2 and component simulations; this is addressed next. Role of warming on sea-ice duration trends The CORE2 simulation differs from the WALL simulation in that: it includes the effects of changes in surface air temperature, relative humidity, downward long- and short-wave radiation and precipitation on the air–ocean and air–ice heat and fresh water fluxes; and; it allows for non-linear interactions between the wind forcing and the heat and fresh water fluxes. To illustrate where air temperature changes might play a role, in Fig. 6a we show the trend in annual mean surface air temperature in the CORE2 simulation over the 1990–2007 period; prominent warming trends are evident in the East Pacific and West Atlantic Oceans. To elucidate the role of surface air temperature, we difference the WALL and CORE2 simulations ( Fig. 6b ). It can be seen that away from the Antarctic Peninsula, the reductions in sea-ice duration in the West Atlantic and East Pacific are associated with warming surface air temperature trends ( Fig. 6b ). In the West Atlantic, if surface warming is included, the declining trend in sea-ice duration is too great ( Fig. 5a ), and the WALL simulation ( Fig. 5f ) agrees better with the observations. In the East Pacific sector, the surface-warming trend helps to amplify the decline in sea-ice duration, and the CORE2 simulation ( Fig. 5a ) better reflects the observed decline in sea-ice duration ( r =0.52, P <0.001; Fig. 5b ). It is interesting to find the WALL simulation with just variability in the wind forcing being more consistent with the observed trends than the CORE2 simulation in all sectors except the East Pacific. This behaviour is consistent with winds being the main driver of Antarctic sea-ice increases [17] . The WALL simulation is also more consistent with the observed increase in Antarctic sea-ice area between 1979 and 2007 than the CORE2 simulation. The better performance of the WALL simulation than CORE2 in four of the sectors may reflect biases in the air temperature trends and errors in the simulated ocean–sea-ice coupling. To assess the robustness of the surface-warming trend, we compute the sea surface-warming trend from two different observationally derived products [33] , [34] ( Fig. 6d,e ). In the East Pacific, the observational sea surface temperature (SST) show a warming trend consistent with the air temperature trend ( Fig. 6a,d,e ). However, in the other sectors the air temperature trends are much larger than the sea surface-warming trends. Substantial air temperature warming trends occur along Antarctica in the West Atlantic, Indian Ocean and Ross Sea that are weak or absent in the SST trends derived from the observational products ( Fig. 6a,d,e ). Fig. 6c shows the simulated SST trend from the CORE2 simulation, which only uses air temperature in its forcing with no additional restoring to sea surface temperature. There is a good correspondence in the simulated SST warming trend and regions where differences in the sea-ice duration trends occur in the WALL–CORE2 simulations. To show air temperature forcing has an important impact on the sea-ice simulation we perform an additional simulation (WALLa) that used all the wind and air-temperature variability from CORE2 in its atmospheric forcings. Using the pattern correlation of the sea-ice duration trends shows for the whole of the Southern Hemisphere, WALLa is well correlated with the CORE2 simulation ( r =0.7), which is greater than the WALL correlation with CORE2 ( r =0.54). In the East Pacific–West Atlantic sector, where the surface-warming trend is greatest, the WALLa simulation shows a greater correlation with the CORE2 simulation ( r =0.76) than the WALL simulation ( r =0.56). The highest correlation between the CORE2 and WALLa simulations occurs in the East Pacific sector ( r =0.84), where we identify warming as playing an important role in the ice trends. While the air temperature makes an important contribution to the difference between the CORE2 and WALL simulations, particularly in the East Pacific, the other atmospheric components of the CORE2 forcing (relative humidity, downward short- and long-wave radiation and precipitation) also play a role in the difference. Further investigation of the role of these terms in the CORE2 forcing needs to be explored. Also, it would be useful to explore the sensitivity of the simulated sea-ice variability and trends to different atmospheric reanalysis products. Sea-ice both responds to and influences our climate [7] ; therefore, understanding sea-ice variability is important for projecting future climate variability and change. Key to gaining such understanding is elucidation of the mechanisms that cause Southern Hemisphere sea-ice to display distinct regional heterogeneity in its interannual variability and trends. By applying separately the interannual and synoptic components of the atmospheric forcing, our study sheds light on how the different atmospheric forcing drives regional sea-ice variability, independent of the usual caveats encountered when applying standard time series analysis methods (empirical orthogonal functions and regressions) to relatively short observational data sets (such as remotely sensed sea-ice data); such analysis is further complicated by how winds can influence sea-ice through both direct and lagged responses [20] . The sea-ice duration trends reflect the combined response to all components of atmospheric forcing and we recognize that the system is non-linear and the response of the full atmospheric forcing is not just the sum of the various components. However, our component simulations help us to identify where weather, ENSO and SAM wind forcing have a significant impact on the trends. We have characterized schematically the trends in sea-ice duration and concentration in various regions around Antarctica according to their response to the atmospheric component forcings. Specifically (see Fig. 7 ), based on comparisons with the observed heterogeneous trends in Antarctic sea-ice duration, the Southern Ocean can be divided into five distinct sectors with the following behaviour. The East Atlantic–West Indian sector exhibits an increase in sea-ice duration where atmospheric weather forcing makes an important contribution while the ENSO contribution is small and the SAM contribution insignificant. In the East Indian sector, there is a weak decrease in sea-ice duration where atmospheric weather forcing makes an important contribution while the contribution from SAM is weak and ENSO is insignificant. For the West Pacific sector there is an increase in sea-ice duration where the SAM and ENSO forcings produce similar increasing trends, while weather forcing produces a weak decreasing trend. In the East Pacific sector there is a strong decrease in sea-ice duration where ENSO forcing produces a similar pattern of decline, but the addition of warming is required for the simulated decrease to be comparable to the observations. In this sector weather forcing produces an increasing duration trend along the Antarctic Peninsula and the SAM forcing produces no trend. The West Atlantic sector shows a decrease in sea-ice duration. In this sector, weather and ENSO forcing produces increasing trends, while the SAM forcing produces no trend. It is only when all wind forcing is combined that the observed decrease in sea-ice duration is simulated. For all sectors, wind forcing makes an important contribution to the recent sea-ice duration trends. Our simulations support analyses of satellite-tracked sea-ice motion for the period 1992–2010, which indicate large and statistically significant trends in Antarctic ice drift in most sectors of the Southern Ocean that are linked, in most regions, to local winds [16] with the added complexity that there may be lagged responses [20] . 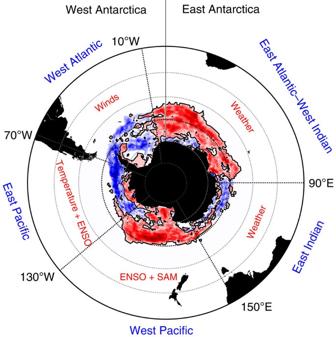Figure 7: Observed trends in sea-ice duration for the 1990–2007 period divided into five distinct regions denoted by the blue text. From the CORE2, ENSO, SAM, WHF and WALL simulations (Fig. 5a,c–f) we identify the dominant forcing mechanisms, indicated by red text, that drive the regional trend in each sector. Figure 7: Observed trends in sea-ice duration for the 1990–2007 period divided into five distinct regions denoted by the blue text. From the CORE2, ENSO, SAM, WHF and WALL simulations ( Fig. 5a,c–f ) we identify the dominant forcing mechanisms, indicated by red text, that drive the regional trend in each sector. Full size image Some of the Antarctic sea-ice trends in the Pacific and Atlantic can be attributed to trends in warming, SAM and ENSO, which could arise through both natural variability and effects due to the Southern Hemisphere ozone hole and increased levels of greenhouse gases [35] . However, the present study provides further evidence that wind forcing influences much of the observed heterogeneity in Antarctic sea-ice. The WALL simulation shows the wind variability other than ENSO, SAM and weather and the potential non-linear interaction of ENSO, SAM and weather forcing have an important impact on the recent trends in winter sea-ice. The WALL simulations show the best agreement with the observed sea-ice duration trends in all sectors but the East Pacific where warming is important. Our simulations show air-temperature variability, particularly in the East Pacific, is an important factor for the differences in sea-ice duration trends between the CORE2 and WALL simulations. However, the downward long and short radiation, relative humidity and precipitation and their potential non-linear interactions with the winds also contribute to the differences between these two simulations. Additional sensitivity studies of the simulated sea-ice variability and trends are needed to explore the individual impacts of downward long and short radiation, relative humidity and precipitation as well as to investigate the robustnesses of the simulation to different atmospheric reanalysis products. It is interesting to note that weather alone can produce trends in sea-ice duration. The ability of synoptic weather to generate multi-decadal trends in sea-ice duration arises through ocean–sea-ice coupling [31] . The recent analysis of mid-latitude tropospheric circulation reveals multi-year variability in the persistence and frequency of atmospheric blocking [36] . Such changes alter synoptic weather and the wind forcing of the ocean by the atmosphere, introducing another way for winds to generate multi-decadal changes in sea-ice. Therefore, in addition to the ways in which the occurrence and strength of SAM [37] , ENSO [38] and ice-sheet melt [39] may change, one must also consider how changes in the synoptic weather patterns may alter the future nature of winter sea-ice in the Southern Hemisphere. Model description The model that we employ for our simulations is the ‘Australian Community Climate Earth System Simulator—Ocean’ (ACCESS—o) configuration of the GFDL MOM4p1 ocean–ice code [40] . Our configuration uses the mass-conserving non-Boussinesq version, involving p * pressure coordinates scaled with height in the vertical direction. To reduce model drift, weak restoring is applied to the salinity of the top layer (with an equivalent thickness of 10 m) by relaxing it to the observed annual mean value [41] over a timescale of 60 days. The model uses an eddy parameterization for the unresolved eddies [42] and the KPP mixing scheme for vertical mixing [43] . ACCESS—o employs a tripolar ocean model grid that has a 360 × 300 logically rectangular horizontal mesh overlying an orthogonal curvilinear grid; a singularity at the north pole is avoided by using a tripolar grid [44] . This approach provides reasonably fine resolution in the Arctic Ocean, while at the same time enhancing computational efficiency. Along the curvilinear zonal direction, ACCESS—o has a regularly spaced grid with 1° resolution. In the meridional direction the grid spacing is nominally 1°, but with the following three refinements: (1) a tripolar Arctic north of 65°N; (2) equatorial refinement to (1/3)° between 10°S and 10°N; (3) a Mercator (cosine-dependent) implementation for the Southern Hemisphere, ranging from 0.25° at 78°S to 1° at 30°S. Sea-ice data The sea-ice concentration data set used was derived from multiple satellite measurements [26] . We use version 2 of the daily data (every other day before July 1987) gridded on to the polar stereographic grid (25 × 25 km) that is available for download from: http://nsidc.org/data/docs/daac/nsidc0079_bootstrap_seaice.gd.html . Vector correlation For the calculation, April–October daily wind and sea-ice drift vectors are averaged into yearly means, and the resulting time series are then correlated at each grid point using a vector correlation [45] . According to the method, the two vector time series are perfectly correlated if the magnitudes of the vectors are related by a constant factor and their directions by a constant offset [45] . The resulting r 2 is scaled to lie between 0 and 1, and we estimate that a correlation of r 2 =0.4 corresponds to a significance level of 99% (ref. 16 ). Experimental design This study employs atmospheric fields from the COREs [46] , [47] for global ocean–ice modelling. For our experimental configuration, we use the CORE version 1 nominal year forcing and the CORE version 2 interannually varying forcing (1948–2007), referred to as CORE1 and CORE2, respectively, which are available from the GFDL MOM4 data sets website ( http://data1.gfdl.noaa.gov/nomads/forms/core.html ). All experiments presented in this study use atmospheric fields, which are then converted to air–sea fluxes with the bulk formulas implemented in MOM4p1 (ref. 43 ). The atmospheric fields used are air temperature, relative humidity, downward short- and long-wave radiation, surface winds and precipitation. The use of bulk formula representations of the heat fluxes [43] , ensure consistent interaction between sea-ice variability and the air–sea heat fluxes. Intrinsic sea-ice variability is simulated using nominal year (CORE1) forcing. A spun-up ocean state was produced by initializing the temperature and salinity fields with World Ocean Atlas [48] , [49] and forcing the model with the CORE1 climatological atmospheric fields, and then running the model until a quasi-steady state is reached where the drift is negligible (1,000 years). From this spun-up state we conducted the experiments summarized below. The simulation was continued for another 100 years using the same CORE1 atmospheric forcing fields; we call this the CORE1 experiment. The last 60 years of this simulation were used to represent the 1948–2007 period for the CORE1 simulation. To investigate the influence of weather, we took the atmospheric winds south of 30°S from the CORE2 data set and high-pass filtered them to remove all variability over durations longer than 1 year. Such filtering removes the interannual variability in the winds but retains the synoptic weather features. North of 30°S we used the winds from CORE1. With the exception of the winds, all other atmospheric forcing fields in this experiment come from CORE1. The simulation with these atmospheric forcing fields was performed for the 1948–2007 period, and the experiment is referred to as WHF. To ensure that the simulation is stable, we repeated the forcing fields for two rounds of the 1948–2007 period and then compared the two sets of results. The two rounds did not produce significant differences in the simulated 1990–2007 sea-ice variability and trends. To investigate low-frequency variability in the CORE2 data due to SAM and ENSO, the monthly zonal winds over the Southern Ocean south of 30°S from the CORE2 data set had their seasonal climatology removed and were reduced to empirical orthogonal functions (EOFs). The first component (21% of the variance) describes the SAM, and a combination of the second and third components (11% and 9% of the variance, respectively) describes the ENSO [31] . The zonal winds in the SAM experiment were constructed by adding a 12-month smoothed first EOF component to the CORE1 winds. North of 30°S the CORE1 winds were used. To assess the consistency of the constructed SAM index (principal component 1), we correlated its 12-month running mean with a 12-month running mean of the SAM index from the NOAA Climate Prediction Center ( www.cpc.ncep.noaa.gov ). Over the 1979–2007 period, the two indices are strongly correlated ( r =0.93). The ENSO zonal winds were constructed by adding 12-month smoothed second and third EOF components to the CORE1 winds. The meridional SAM and ENSO components of the winds for south of 30°S were constructed by regressing the monthly zonal winds of SAM and ENSO, respectively, on the CORE2 monthly meridional winds with the seasonal climatology removed. These two zonal wind products were then added to the CORE1 winds to get the SAM and ENSO meridional winds. For the other atmospheric fields, both these experiments used the CORE1 fields. The SAM and ENSO forcing simulations were run both separately and as a combined simulation (ENSO+SAM). Each of the SAM, ENSO and ENSO+SAM simulations were performed for two rounds of the 1947–2007 period, and we report the results from the second round. Like the WHF simulation, for all these simulations there were no significant differences between the two rounds of forcing in the sea-ice variability and trends over the 1990–2007 period. To assess the role of wind variability an experiment was conducted that used global CORE2 winds together with CORE1 fields for the other atmospheric forcing fields. Thus, the experiment retains all the wind variability, and hence is referred to as WALL, but is forced only by the seasonal climatology for air temperature, relative humidity, downward short- and long-wave radiation, and precipitation. The WALL simulation was performed for two rounds of the 1947–2007 period, with results from the second round reported in this paper. Like experiments 2–4, we found no significant differences between the two rounds of forcing in the sea-ice variability and trends for the 1990–2007 period. To assess the role of wind and air-temperature variability a final experiment was conducted based on the WALL forcing but using the CORE2 air temperature in its forcing (WALLa) rather than the CORE1 fields. The complete set of experiments and their acronyms are summarized in Table 1 . In all experiments except CORE2 and WALLa, only the winds are changed, and the other atmospheric fields required by the bulk formula parameterization of the air–sea fluxes use the CORE1 seasonal climatologically varying atmospheric fields. In the CORE2 experiment, all atmospheric fields are interannually varying. In the WALLa experiment only the winds and air temperatures vary interannually. As an example of the difference in wind forcing between CORE1 and CORE2 we show the winds of 1 April 1995 ( Fig. 8 ). We can make this direct comparison in 1995 because CORE1 winds are based on 1995 with additional processing at each grid point in the wind fields to ensure the spectra of CORE1 variability matches the CORE2 spectra [46] . While the CORE1 winds have similar synoptic features, the difference between CORE2 and CORE1 shows many small-scale features. These small-scale features introduce spatial noise into the CORE1 winds, which substantially changes the ocean and sea-ice variability [30] . 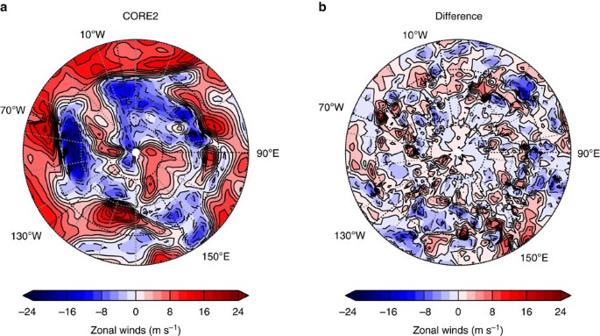Figure 8: Zonal wind field for 1 April 1995. Used in the (a) WHF simulation; and (b) the difference in the zonal wind field between WHF and CORE1 simulations. Figure 8: Zonal wind field for 1 April 1995. Used in the ( a ) WHF simulation; and ( b ) the difference in the zonal wind field between WHF and CORE1 simulations. Full size image Code availability The combined ocean sea-ice model code used in this study is based on the GFDL MOM4p1 code. The code we used along with the namelist file (input.nml) and the run-time configuration file (field_table) are archived and available at http://www.marine.csiro.au/mat236/ice.tar . How to cite this article: Matear, R. J. et al . Sources of heterogeneous variability and trends in Antarctic sea-ice. Nat. Commun. 6:8656 doi: 10.1038/ncomms9656 (2015).